Iron-catalysed transformation of molecular dinitrogen into silylamine under ambient conditions Although stoichiometric transformations using transition metal–N 2 complexes have been well investigated towards the goal of nitrogen fixation under mild reaction conditions, only a few examples of the catalytic transformations of N 2 using transition metal–N 2 complexes as catalysts have been reported. In almost all the catalytic systems, the use of Mo is essential to realize the catalytic transformation of N 2 , where Mo–N 2 complexes are considered to work as effective catalysts. Here we show the first successful example of the Fe-catalysed transformation of N 2 into N(SiMe 3 ) 3 under ambient conditions, in which iron complexes such as iron pentacarbonyl [Fe(CO) 5 ] and ferrocenes have been found to work as effective catalysts. A plausible reaction pathway is proposed, where Fe(II)–N 2 complex bearing two Me 3 Si groups as ancillary ligands has an important role as a key reactive intermediate, with the aid of density-functional-theory calculations. Nitrogen fixation, the production of ammonia (NH 3 ) from N 2 , is one of the most important processes for our continued survival as NH 3 is widely used as an essential source of nitrogen fertilizer. However, N 2 is regarded as one of the most inert molecules, which hardly undergoes chemical transformation under usual reaction conditions. Industrially, NH 3 is produced from N 2 and H 2 using Fe-based heterogeneous catalysts under harsh reaction conditions, where enormous energy is also necessary for the production of H 2 from fossil fuels such as natural gas [1] . Although the stoichiometric transformation using transition metal–N 2 complexes has been well investigated towards the goal of nitrogen fixation under mild reaction conditions [2] , [3] , [4] , only a few examples of the catalytic transformation of N 2 using transition metal–N 2 complexes [5] , [6] as catalysts have been reported [7] , [8] , [9] . In fact, only two types of Mo–N 2 complexes bearing triamidoamine [7] ligand and 2,6-bis(di-tert-butylphosphinomethyl)pyridine [9] ligand, respectively, worked as effective catalysts to promote the direct conversion of N 2 into NH 3 under ambient reaction conditions. The method for the catalytic formation of N(SiMe 3 ) 3 (1) from N 2 has been known as an alternative nitrogen fixation route because 1 is quantitatively converted to NH 3 upon hydrolysis. The first example of the catalytic formation of 1 was reported for the reaction of N 2 with Li as a reducing agent and Me 3 SiCl in the presence of various metal salts, such as CrCl 3 as catalysts, where up to 5.4 equiv. of 1 was produced based on the catalyst [10] . In this reaction system, the possibility of the formation of lithium nitride (Li 3 N) as a reactive intermediate cannot be completely excluded (similarly, Mori [11] also reported the transformation of N 2 using Li as a reducing agent in the presence of Ti complexes). Later, the Mo-catalysed conversion of N 2 into 1 using Na as a reducing agent was reported by Hidai and co-workers [12] , where up to 24 equiv. of 1 was produced based on the catalyst. More recently, we have found a more efficient catalytic system using a Mo–N 2 complex bearing two ferrocenyldiphosphines as a key catalyst, where up to 226 equiv. of 1 was produced based on the catalyst, and have proposed a possible reaction pathway based on density-functional-theory (DFT) calculations [13] . In almost all the catalytic systems mentioned above, the use of Mo in the catalyst is essential to realize the catalytic transformation of N 2 under ambient conditions, where Mo–N 2 complexes are considered to work as effective catalysts. As an extension of our study [13] , [14] , [15] , we now report the Fe-catalysed reduction of N 2 into 1 under ambient conditions, where up to 34 equiv. of 1 was produced based on the catalyst. In this reaction system, simple and commercially available Fe complexes such as [Fe(CO) 5 ] and ferrocenes have been found to work as effective catalysts. This is the first successful example of the Fe-catalysed conversion of N 2 under ambient conditions. An Fe–N 2 complex bearing two Me 3 Si ligands has been proposed to work as a key reactive intermediate following DFT calculations on the real reaction system. Iron-catalysed reaction of N 2 into N(SiMe 3 ) 3 The catalytic reduction of N 2 into 1 using [Fe(CO) 5 ] (0.10 mmol) as a catalyst was investigated according to the following procedure. A mixture of Na (600 equiv. to the Fe atom in the catalyst), Me 3 SiCl (600 equiv. to the Fe atom in the catalyst) and [Fe(CO) 5 ] in tetrahydrofuran (THF) (40 ml) was stirred at room temperature for 20 h under 1 atm of N 2 . After the reaction, 1 (25 equiv. to the Fe atom in the catalyst) was revealed to be formed together with other trimethylsilylated compounds such as hexamethyldisilane ( 2 ), butoxytrimethylsilane ( 3 ) and trimethyl(4-(trimethylsilyl)butoxy)silane ( 4 ) (see Supplementary Table S1 ). The scheme for the catalytic formation of 1 is shown in Fig. 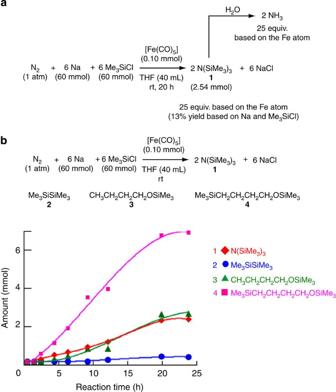Figure 1: Catalytic reaction of N2into N(SiMe3)3(1) in the presence of a catalytic amount of [Fe(CO)5] (a) [Fe(CO)5]-catalysed formation of N(SiMe3)3(1) from N2(1 atm) at room temperature (rt) for 20 h in THF. (b) Time profile of the reaction of N2(1 atm) with Na and Me3SiCl in the presence of a catalytic amount of [Fe(CO)5] at rt in THF. 1a , and typical results are summarized in Table 1 . Separately, we confirmed that the produced 1 can be readily converted into NH 3 quantitatively (25 equiv. to the Fe atom in the catalyst) after hydrolysis of the crude reaction mixture. The present method for the formation of 1 is considered to provide a direct approach to produce NH 3 equivalent from N 2 under ambient conditions. Figure 1: Catalytic reaction of N 2 into N(SiMe 3 ) 3 (1) in the presence of a catalytic amount of [Fe(CO) 5 ] ( a ) [Fe(CO) 5 ]-catalysed formation of N(SiMe 3 ) 3 ( 1 ) from N 2 (1 atm) at room temperature (rt) for 20 h in THF. ( b ) Time profile of the reaction of N 2 (1 atm) with Na and Me 3 SiCl in the presence of a catalytic amount of [Fe(CO) 5 ] at rt in THF. Full size image Table 1 Catalytic reaction of N 2 into N(SiMe 3 ) 3 ( 1 ) in the presence of a catalytic amount of Fe catalyst*. Full size table The amount of 1 did not increase even for a longer reaction time such as 100 h. When the catalytic reaction was carried out at a higher reaction temperature, such as 60 °C for 20 h, the amount of 1 slightly decreased, where 16 equiv. amount of 1 were produced based on the Fe atom. In the reaction with Li as a reducing agent in place of Na, only a small amount of 1 was formed together with a large amount of 2 . The use of other polar and non-polar solvents such as diethyl ether, 1,4-dioxane, 1,2-dimethoxyethane, benzene and hexane were not effective for the present catalytic reaction. Separately, we confirmed that no formation of 1 was observed in the absence of N 2 (under argon atmosphere) or [Fe(CO) 5 ]. These results indicate that [Fe(CO) 5 ] in THF worked as an effective catalyst for the formation of 1 from N 2 . When bis(trimethylsilyl)iron tetracarbonyl complex [Fe(SiMe 3 ) 2 (CO) 4 ] (ref. 16 ) was used in place of [Fe(CO) 5 ], a slightly larger amount of 1 (29 equiv.) was produced under similar reaction conditions. Some other iron carbonyl complexes bearing a cyclopentadienyl moiety such as cyclopentadienyliron dicarbonyl dimer [CpFe(CO) 2 ] 2 (Cp=η 5 -C 5 H 5 ) also worked as catalysts, where a slightly smaller amount of 1 was produced based on the Fe atom of the catalyst. Interestingly, a simple and historic iron complex, ferrocene [Cp 2 Fe], also worked as a catalyst towards the formation of 1 under similar reaction conditions, although slightly less effectively. Here the introduction of Me 3 Si moieties to the cyclopentadienyl ring of the ferrocene as electron-withdrawing groups to the aromatic rings substantially improved the catalytic activity. In fact, 1,1′,2,2′,4,4′-hexakis(trimethylsilyl)ferrocene [{η 5 -C 5 H 2 (SiMe 3 ) 3 } 2 Fe] (ref. 17 ) worked as the most effective catalyst, where the largest amount of 1 (34 equiv.) was produced based on the Fe atom in the catalyst. In sharp contrast, the introduction of alkyl groups, such as methyl and butyl moieties, at the cyclopentadienyl ring of the ferrocene [(η 5 -C 5 H 4 R) 2 Fe] (R=Me, t Bu) dramatically decreased the amount of 1 . It is noteworthy that iron salts such as FeCl 2 and [Fe{N(SiMe 3 ) 2 } 2 ] did not work as effective catalysts under the present reaction conditions. Time profile of iron-catalysed reaction of N 2 into N(SiMe 3 ) 3 In order to obtain more information on the reaction pathway, the relationship between the reaction time and the yields of 1 was investigated in the reaction of N 2 (1 atm) with Na and Me 3 SiCl in the presence of a catalytic amount of [Fe(CO) 5 ] in THF at room temperature. The time profile is shown in Fig. 1b . An induction period (ca. 1 h) was observed at first, probably because of the formation of an active Fe catalyst. Then, the formation of 1 proceeded until 20 h parallel to that of other trimethylsilylated compounds, such as 2 , 3 and 4 . No further formation of all products was observed after 20 h. These results indicate that 2 , 3 and 4 were produced simultaneously together with 1 . Next, we would like to discuss Fe species serving as catalysts in our reaction systems, although unfortunately, no Fe–N 2 species have yet been isolated and identified from the reaction mixture. Our speculation will be logically supported by some experimental findings with the aid of quantum chemical calculations. First, we have investigated the catalytic reaction in the presence of a large excess amount of Hg as mercury-poison test [18] . However, no influence of Hg was observed at all. As a result, we removed the possibility that Fe nanoparticles generated in situ work as true active species in the present reaction system. This result apparently indicates that the catalytic active species is a homogeneous Fe complex. Second, the experimental result that both [Fe(CO) 5 ] and ferrocenes have almost the same catalytic activity towards the formation of 1 suggests that common Fe complexes, generated in situ from Na, Me 3 SiCl and Fe species, work as real catalysts. Third, for the formation of 1 catalysed by a Mo–N 2 complex, we have already proposed a reaction mechanism, where a Me 3 Si radical has an important role to promote the catalytic reduction of N 2 (ref. 13 ). It should be stressed that [Fe(SiMe 3 ) 2 (CO) 4 ] (ref. 16 ) worked as one of the most effective catalysts towards the formation of 1 . The reaction of [Na 2 Fe(CO) 4 ], prepared from [Fe(CO) 5 ] and Na, with Me 3 SiCl has been known to give [Fe(SiMe 3 ) 2 (CO) 4 ], whereas the reactions of ferrocene with reducing agents have recently been reported to give the corresponding low-valent Fe(0 or -II) complexes [19] , [20] , which may be easily converted into the Fe(II)(SiMe 3 ) 2 species by treatment with Me 3 SiCl and/or Me 3 Si radical. These results indicate that two Me 3 Si groups can readily be introduced to the Fe atom of the Fe complexes under the catalytic conditions. For the reasons listed above, we propose [Fe(II)(SiMe 3 ) 2 (THF)] ( I ) and [Fe(II)(SiMe 3 ) 2 Cl] − ( I′ ) as the common catalysts in our reaction systems. Optimized geometries of I and I′ are depicted in Fig. 2 . In fact, their Fe(II) analogues, such as [Fe{Si(SiMe 3 ) 3 } 2 (THF)] [21] and [Fe{Si(SiMe 3 ) 3 } 2 Cl] − (ref. 22 ), have been prepared and characterized spectroscopically. Recently, Fe–N 2 complexes bearing two silyl ligands [(η 6 -arene) Fe(Me 2 SiC 6 H 4 SiMe 2 )] 2 (μ-η 1 :η 1 -N 2 ) have been prepared and characterized by X-ray analysis [23] . 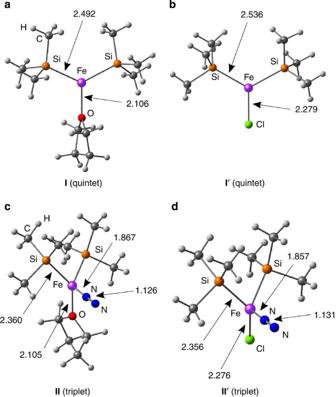Figure 2: Molecular structures optimized at the B3LYP*/6-311+G** level of theory. Bond distances are presented in Å (a) [Fe(SiMe3)2(THF)] (I). (b) [Fe(SiMe3)2Cl]−(I′). (c) [Fe(SiMe3)2(N2)(THF)] (II). (d) [Fe(SiMe3)2(N2)Cl]−(II′). Figure 2: Molecular structures optimized at the B3LYP*/6-311+G** level of theory. Bond distances are presented in Å ( a ) [Fe(SiMe 3 ) 2 (THF)] ( I ). ( b ) [Fe(SiMe 3 ) 2 Cl] − ( I′ ). ( c ) [Fe(SiMe 3 ) 2 (N 2 )(THF)] ( II ). ( d ) [Fe(SiMe 3 ) 2 (N 2 )Cl] − ( II′ ). Full size image In order to examine the N 2 -activating ability of I and I′ , we have performed DFT calculations on the corresponding N 2 complexes [Fe(SiMe 3 ) 2 (N 2 )(THF)] ( II ) and [Fe(SiMe 3 ) 2 (N 2 )Cl] − ( II′ ). Optimized geometries of II and II′ depicted in Fig. 2 adopt a slightly deformed tetrahedral structure. The Fe–N 2 bond energy of II (12.1 kcal mol −1 ) is higher than that of II′ (7.7 kcal mol −1 ). The N–N bond distance (the N–N stretching frequency) is 1.126 Å (2,122 cm −1 ) for II and 1.131 Å (2,082 cm −1 ) for II′ . The coordinated N 2 on the Fe atom is moderately activated relative to free N 2 (1.098 Å (2,422 cm −1 )), although the calculated Fe–N 2 bond energies suggest that II and II′ are hard to be isolated experimentally. Based on the results of catalytic reaction and the calculations on the Fe–N 2 complexes, we propose the reaction pathway for catalytic transformation of N 2 into 1 as shown in Fig. 3 . At first, a Fe(II)–N 2 complex bearing two Me 3 Si groups, such as II , is formed via I , which generated in situ Na, Me 3 SiCl and Fe species ( vide supra ). A sequential addition of three Me 3 Si radicals to the distal N atom of the coordinated N 2 ligand in II proceeds to form [Fe(IV)(SiMe 3 ) 2 (THF)(NN(SiMe 3 ) 3 )] ( A ). The N–N bond cleavage of the complex A occurs to afford the first molecule of 1 together with the formation of [Fe(II)(SiMe 3 ) 2 (N(SiMe 3 ) 3 )(THF)] ( B ) after the addition of further three Me 3 Si radicals. Finally, the complex B liberates the second molecule of 1 to regenerate the starting complex I . We have theoretically confirmed that this catalytic mechanism is reasonable by assuming I as the catalyst (see Supplementary Figs S2–S10 and Supplementary Tables S4–S34 ). 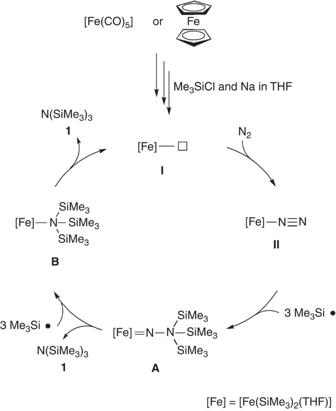Figure 3: A proposed reaction pathway. The pathway is supported by the DFT calculations, where Fe–N2complex is capable of serving as a suitable catalyst for the conversion of N2into N(SiMe3)3(1). Figure 3: A proposed reaction pathway. The pathway is supported by the DFT calculations, where Fe–N 2 complex is capable of serving as a suitable catalyst for the conversion of N 2 into N(SiMe 3 ) 3 ( 1 ). Full size image In summary, we have found some iron complexes such as iron pentacarbonyl [Fe(CO) 5 ] and ferrocenes work as effective catalysts for the formation of tris(trimethylsilyl)amine (N(SiMe 3 ) 3 ), which is readily converted into NH 3 , from the reaction of molecular dinitrogen (N 2 ) with Na as a reducing agent and trimethylsilyl chloride (Me 3 SiCl) under ambient conditions. In this reaction system, up to 34 equiv. of N(SiMe 3 ) 3 have been produced based on the Fe atom of the catalyst. This is the first successful example of the Fe-catalysed transformation of N 2 into N(SiMe 3 ) 3 under ambient conditions. Two possible Fe(II)-N 2 complexes bearing two Me 3 Si groups as ancillary ligands have been proposed as a key reactive intermediate in the catalytic cycle. Recently, the preparation of Fe–N 2 complexes and their stoichiometric reactivity have been intensively studied [24] , [25] , [26] , [27] , but the Fe-catalysed transformation of N 2 by using Fe–N 2 complexes has not yet been reported until now [28] . We believe that the results described here provide valuable and useful information to develop the Fe-catalysed transformation of N 2 . Further work is currently under way to develop more effective Fe catalysts and the isolation and characterization of reactive intermediates in the catalytic reaction. A typical procedure for catalytic reduction of N 2 into N(SiMe 3 ) 3 To a suspension of sodium (1.38 g, 60 mmol) in THF (40 ml) were added Me 3 SiCl (7.6 ml, 60 mmol) and Fe(CO) 5 (13.2 μl, 0.10 mmol) under dinitrogen atmosphere. The mixture was stirred at room temperature (22–24 °C) for 20 h under a gentle stream of dinitrogen. To the reaction mixture was added cyclododecane (0.100 g) as an internal standard for gas–liquid chromatography (GLC) analysis. After stirring for 5 min, the mixture was centrifuged to remove insoluble materials. The resultant clear supernatant was subjected to GLC and capillary gas chromatography mass spectrometry analyses. Then the supernatant was stirred with an aqueous solution of H 2 SO 4 (0.5 M, 10 ml) for 12 h. After the addition of an aqueous solution of KOH (30 wt %, 10 ml), NH 3 was distilled into an aqueous solution of H 2 SO 4 (0.5 M, 10 ml) under reduced pressure. The amount of NH 3 was determined by the indophenol method. Separately, we confirmed that the following Fe complexes such as [(η 5 -C 5 H 4 R) 2 Fe] (R=Me, t Bu), FeCl 2 and [Fe{N(SiMe 3 ) 2 } 2 ] did not work as effective catalysts under the same reaction conditions. See Supplementary Tables S1 and S2 . Time profile of catalytic formation of N(SiMe 3 ) 3 from N 2 To a suspension of sodium (1.38 g, 60 mmol) in THF (40 ml) were added Me 3 SiCl (7.6 ml, 60 mmol), Fe(CO) 5 (13.2 μl, 0.10 mmol) and cyclododecane (0.102 g) under dinitrogen atmosphere. The mixture was stirred at room temperature under a gentle stream of dinitrogen. An aliquot of the reaction mixture was periodically analysed by GLC. See Supplementary Table S3 . Computational methods DFT calculations were performed to search all intermediates and transition structures on potential energy surfaces by using the Gaussian 09 program [29] . Because the relative energy of different spin states was found to be of great importance in the present monoiron system, we adopted the B3LYP* functional, [30] , [31] , [32] which is a reparametrised version of the B3LYP hybrid functional [33] , [34] developed by Reiher et al. [30] , [31] The B3LYP functional is known to be reliable when applied for molecular and enzymatic systems containing transition metals, but it tends to overestimate the spin-state splitting [35] , [36] , [37] , [38] . Advantages of the B3LYP* functional in the evaluation of the spin-state splitting have been reported for several iron complexes exhibiting spin-crossover phenomena [30] , [31] , [32] , [39] . The B3LYP and B3LYP* energy expression is shown in equation (1): where a 0 =0.20 (B3LYP) or 0.15 (B3LYP*), a x =0.72, a c =0.81; and in which E X HF is the Hartree–Fock exchange energy; E X LSDA is the local exchange energy from the local spin density approximation; E X B88 is Becke’s gradient correction [40] to the exchange functional; E C LYP is the correlation functional developed by Lee et al. [41] ; and E C VMN is the correlation energy calculated using the local correlation functional of Vosko et al. [42] The 6-311+G** basis set was employed for all atoms throughout the present work. Systematic vibrational analyses were carried out for all reaction species to characterize stationary-point structures. An appropriate connection between a reactant and a product for each reaction step was confirmed by intrinsic reaction coordinate (IRC) [43] , [44] , [45] and quasi-IRC calculations. In the quasi-IRC calculation, the geometry of a transition state was at first shifted by perturbing the geometries very slightly along the reaction coordinate and released for equilibrium optimization. The energy profile of the proposed catalytic cycle in Supplementary Fig. S2 is presented using the SCF energies with the zero-point energy correction. In the present reaction system, Me 3 Si radical is a possible active silyl species. The formation of Me 3 Si radical in the presence of sodium in THF (solvent) is theoretically deduced in elsewhere. [13] How to cite this article: Yuki, M. et al. Iron-catalysed transformation of molecular dinitrogen into silylamine under ambient conditions. Nat. Commun. 3:1254 doi: 10.1038/ncomms2264 (2012).